Auxin transport and activity regulate stomatal patterning and development Stomata are two-celled valves that control epidermal pores whose spacing optimizes shoot-atmosphere gas exchange. They develop from protodermal cells after unequal divisions followed by an equal division and differentiation. The concentration of the hormone auxin, a master plant developmental regulator, is tightly controlled in time and space, but its role, if any, in stomatal formation is obscure. Here dynamic changes of auxin activity during stomatal development are monitored using auxin input (DII-VENUS) and output (DR5:VENUS) markers by time-lapse imaging. A decrease in auxin levels in the smaller daughter cell after unequal division presages the acquisition of a guard mother cell fate whose equal division produces the two guard cells. Thus, stomatal patterning requires auxin pathway control of stem cell compartment size, as well as auxin depletion that triggers a developmental switch from unequal to equal division. Stomatal development includes an early stem cell phase followed by symmetric division and differentiation. The former includes the selection and unequal division of a founder stem cell (meristemoid mother cell, MMC), and then the acquisition of a pre-stomatal fate by the smaller cell (meristemoid, M). The larger sister cell of an unequal division, a stomatal lineage ground cell (SLGC), either differentiates into a generic epidermal cell or reacquires a stem cell fate and produces a ‘satellite’ M after unequal division. The M converts to a guard mother cell (GMC) that divides equally followed by a coordinated morphogenesis yielding the two guard cells (GCs) of the stoma [1] , [2] , [3] . The first gene identified as a key regulator of stomatal distribution and patterning was TOO MANY MOUTHS ( TMM ), which encodes a leucine-rich repeat receptor (LRR)-like protein that lacks a cytoplasmic kinase domain. Mutations in TMM induce pattern violations in the form of excess stomata in direct contact [4] , [5] . Along with TMM, ERECTA-family LRR receptor-like kinases perceive secreted peptide ligands [6] , [7] . For example, the epidermal patterning factor (EPF)2 and EPF1 ligands, which are members of the EPF/EPF-like family, are specifically and respectively expressed in early- and late-stage stomatal precursor cells. Loss-of-function epf2 or epf1 mutants display extra stem cells or clustered stomata [8] , [9] , [10] . Auxin widely regulates plant development, such as by coordinating the placement and patterning of organs and cells. Plants have thus evolved complex spatiotemporal mechanisms controlling auxin homoeostasis [11] , [12] , [13] . The key mechanism among these is the active and polar cell-to-cell transport of auxin that is mediated by PIN-FORMED (PIN) proteins and by homologues of ABCB multiple drug resistance transporters [14] , [15] , [16] . Despite the central role of stomata in plant evolution and productivity and their ubiquity throughout the shoot, the role of auxin in stomatal development is incompletely understood. Here we show that stomatal patterning requires auxin pathway control of stem cell compartment size, as well as auxin depletion for switch from unequal to equal division during stomatal development. Auxin activity levels change during stomatal development Stomata arise via unequal divisions of stem cells whose frequency and placement regulates stomatal number, density and their minimal-one-celled separation pattern ( Fig. 1a–c ). On the basis of their patterns of expression, multiple PIN proteins probably function in stomatal development ( Supplementary Fig. 1 ). Membrane-associated fluorescence from a PIN3-GFP (green fluorescent protein) translational fusion [17] is especially strong around two types of stomatal precursor cells, Ms and GMCs. Fluorescence from pPIN3:PIN3-GFP co-localizes with that from FM4-64 that marks the cell membrane [18] ( Supplementary Fig. 2a,b ). For example, fluorescence intensity profiles from PIN3-GFP and FM4-64 were quantified along a transect that included a M and its larger sister cell as well as pavement cells. PIN3-GFP fluorescence from a M was found to be higher than its larger sister cell, a SLGC ( Supplementary Fig. 2c ). This circumferential pattern of PIN fluorescence contrasts with other cell types, such as those in roots, where fluorescence is in the membrane and is often polarized at one end of the cell [14] . Thus, PIN3-GFP signal from Ms and GMCs, like FM4-64, is evenly distributed throughout the cell membrane ( Supplementary Fig. 2d ). PIN3-GFP signal is notably absent from mature GCs ( Supplementary Fig. 2e–g ). 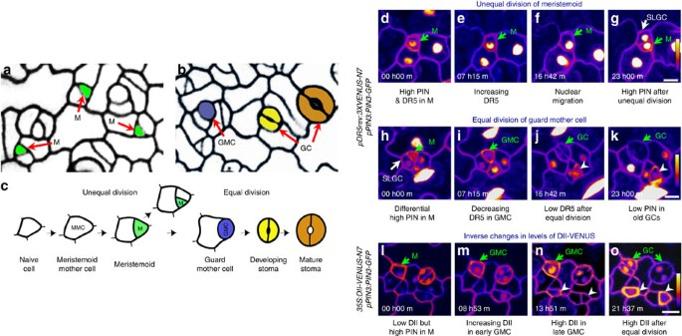Figure 1: Differential PIN3 and auxin activity levels during equal and unequal divisions in stomatal development. (a) Cell outlines in epidermal fields (walls visualized with PI fluorescence). Meristemoids (M, indicated by red arrows), like the stomata they produce, are usually separated by at least one intervening cell, and originate from an unequal division. (b) Each M develops into a guard mother cell (GMC) that in turn produces two guard cells (GCs). (c) Diagram of stomatal development. Unequal divisions generate Ms, while equal divisions of GMCs yield paired GCs. (d) A M is indicated by a green arrow. (e) DR5 level slightly increases in a M. (f) The nucleus migrates to a corner first before unequal division. (g) DR5 and PIN3 levels are comparable in a newly formed M and its larger sister cell, which is a stomatal lineage ground cell (SLGC; white arrow). (h) PIN3 fluorescence is brighter around the M compared with its sister cell, a SLGC. (i) DR5 levels drop strongly in GMCs. (j) Two young GCs after GMC division. (k) DR5 and PIN3 are barely detectable in mature GCs. Arrowhead, a new M forms away from pre-existing GC (j,k). (l) DII fluorescence level is low in a M. (m) DII levels increase at the M to GMC transition. (n) The DII level is high in a GMC just before it divides equally. (o) DII levels remain high in GCs, a sequence opposite to that of DR5. DII levels are low during unequal division (arrowheads innando). Heat map images converted from time-lapse series. Nuclear fluorescence ind–kfrompDR5rev:3XVENUS-N7and inl–ofrom35S:DII-VENUS-N7; membrane fluorescence ind–ofrompPIN3:PIN3-GFP. Vertical colour bars at right indicate intensity range. Numbers at bottom indicate elapsed time. Scale bar, 10 μm. Figure 1: Differential PIN3 and auxin activity levels during equal and unequal divisions in stomatal development. ( a ) Cell outlines in epidermal fields (walls visualized with PI fluorescence). Meristemoids (M, indicated by red arrows), like the stomata they produce, are usually separated by at least one intervening cell, and originate from an unequal division. ( b ) Each M develops into a guard mother cell (GMC) that in turn produces two guard cells (GCs). ( c ) Diagram of stomatal development. Unequal divisions generate Ms, while equal divisions of GMCs yield paired GCs. ( d ) A M is indicated by a green arrow. ( e ) DR5 level slightly increases in a M. ( f ) The nucleus migrates to a corner first before unequal division. ( g ) DR5 and PIN3 levels are comparable in a newly formed M and its larger sister cell, which is a stomatal lineage ground cell (SLGC; white arrow). ( h ) PIN3 fluorescence is brighter around the M compared with its sister cell, a SLGC. ( i ) DR5 levels drop strongly in GMCs. ( j ) Two young GCs after GMC division. ( k ) DR5 and PIN3 are barely detectable in mature GCs. Arrowhead, a new M forms away from pre-existing GC ( j , k ). ( l ) DII fluorescence level is low in a M. ( m ) DII levels increase at the M to GMC transition. ( n ) The DII level is high in a GMC just before it divides equally. ( o ) DII levels remain high in GCs, a sequence opposite to that of DR5. DII levels are low during unequal division (arrowheads in n and o ). Heat map images converted from time-lapse series. Nuclear fluorescence in d – k from pDR5rev:3XVENUS-N7 and in l – o from 35S:DII-VENUS-N7 ; membrane fluorescence in d – o from pPIN3:PIN3-GFP . Vertical colour bars at right indicate intensity range. Numbers at bottom indicate elapsed time. Scale bar, 10 μm. Full size image Fluorescence from pPIN3:PIN3-GFP and from the synthetic auxin-responsive reporter pDR5rev:3XVENUS-N7 (ref. 19 ), which localized to the cell membrane and nucleus, respectively ( Supplementary Movie 1 ), were tracked during stomatal development using in vivo time-lapse confocal microscopy ( Supplementary Fig. 3 and Supplementary Movie 2 ). DR5:VENUS and PIN3-GFP fluorescence levels are moderate around the time of unequal division and are roughly equal in nascent daughter cells ( Fig. 1d–g ). After unequal division, the M is differentially brighter in PIN3-GFP fluorescence compared with its larger sister cell ( Fig. 1g,h ). Nuclear-localized DR5:VENUS levels in the M progressively decrease >1.5 times before the GMC divides equally ( Fig. 1h,i and Supplementary Table 1 ). DR5:VENUS levels drop further after this division, with only faint fluorescence present in mature GCs ( Fig. 1j,k ). Auxin stabilizes interactions between the auxin co-receptor SCF TIR1/AFB1-5 and Aux/IAAs proteins, thereby driving proteasomal degradation of Aux/IAAs, which in turn increases the availability of auxin response factors (ARFs) to regulate the transcription of auxin response genes [20] . Changes in auxin signalling input activity were tracked through time using DII-VENUS whose fluorescence correlates inversely with that of DR5, which is a proxy for cellular auxin transcriptional output signalling [21] . DII-VENUS signals increased during the M to GMC developmental transition indicating reduced signal input at the GMC stage ( Fig. 1l–o , and Supplementary Fig. 4 and Supplementary Movie 3 ). The absence of DII-VENUS signal from unequal divisions is consistent with high levels of auxin in precursor cells inducing DII degradation ( Fig. 1n,o ; arrowheads). Together, these (inverse) changes in DII-VENUS and DR5:VENUS fluorescence levels demonstrate reduced cellular auxin signalling activity (input and output, respectively) during the M to GMC developmental transition. Auxin efflux is required for stomatal patterning and number Stomata are separated by at least one intervening cell [1] , [3] . To determine whether this spacing involves PIN protein-mediated auxin transport, loss-of-function mutants in each PIN gene were examined, but none showed any stomatal defects. However, in contrast to the spaced stomata in wild types ( Fig. 2a ), two different quadruple mutants, pin2, 3, 4, 7 ( Fig. 2b ) and pin1, 3, 4, 7 ( Supplementary Fig. 5a ) displayed pattern defects in the form of groups of stomata in direct contact (around 20% stomata in clusters), indicating functional redundancy between PINs, which is consistent with the expression of multiple PINs in the epidermis ( Supplementary Fig. 1 ). Weak patterning defects were found in a pin1, 4, 7 triple mutant (about 6% of stomata were clustered), indicating a requirement of PIN3 in stomatal pattering. A similar defect occurred in mutants in PINOID, which encodes a protein kinase that mediates the targeting of multiple PINs to the cell membrane [22] , [23] ( Supplementary Fig. 5b ). The gene most closely related to PIN3 is PIN7 (ref. 24 ) but the latter is not normally expressed in the stomatal lineage. However, PIN7-GFP signal is slightly enhanced in cells outside the stomatal lineage in a pin3-4 mutant consistent with compensatory functional redundancy between PINs in epidermal cells (similar to roots and embryos [24] ) ( Supplementary Fig. 6 ). Stomatal patterning thus probably requires PIN-mediated transport of auxin. However, stomatal phenotypic defects are also present in tir1, afb1, 2, 3 quadruple mutants [25] , [26] , thus reinforcing the involvement of auxin signalling in stomatal patterning ( Fig. 2c and Supplementary Fig. 5 ). 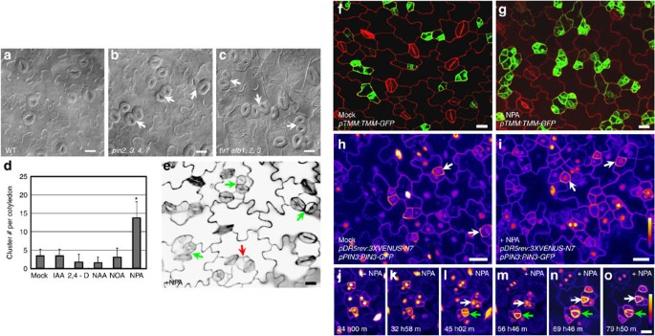Figure 2: Modulated auxin efflux is required for stomatal patterning and number. (a) A wild-type epidermis. (b) Abnormal stomatal clusters form in apin2, 3, 4, 7quadruple mutant. (c) Clusters form in atir1 afb1, 2, 3quadruple mutant. (d) Stomata in contact arise when auxin efflux is inhibited by NPA, but not by exogenous auxin, IAA or NAA, 2,4-dichlorophenoxyacetic acid (2,4-D) or by the auxin influx inhibitor 1-naphthoxyacetic acid (NOA). (e) NPA-treated wild-type epidermis showing stomata in contact (green arrows) and an ectopic unequal division (red arrow). (f) Fluorescence frompTMM:TMM-GFP.(g) NPA induces abnormal groups of stem cells in contact that expresspTMM:TMM-GFP. (h) Heat map images ofpPIN3:PIN3-GFPandpDR5rev:3XVENUS-N7in epidermis after dimethylsulphoxide (DMSO; mock) treatment. (i) NPA increases nuclear DR5 fluorescence in GMCs (arrows). (j–o) Time-lapse series showing NPA-induced excess unequal divisions in wild type. NPA significantly slows the decline of DR5 fluorescence in a new M (a white arrow); however, a M with high PIN3 levels progresses normally to stomatal differentiation (a green arrow). Scale bar, 10 μm. Figure 2: Modulated auxin efflux is required for stomatal patterning and number. ( a ) A wild-type epidermis. ( b ) Abnormal stomatal clusters form in a pin2, 3, 4, 7 quadruple mutant. ( c ) Clusters form in a tir1 afb1, 2, 3 quadruple mutant. ( d ) Stomata in contact arise when auxin efflux is inhibited by NPA, but not by exogenous auxin, IAA or NAA, 2,4-dichlorophenoxyacetic acid (2,4-D) or by the auxin influx inhibitor 1-naphthoxyacetic acid (NOA). ( e ) NPA-treated wild-type epidermis showing stomata in contact (green arrows) and an ectopic unequal division (red arrow). ( f ) Fluorescence from pTMM:TMM-GFP. ( g ) NPA induces abnormal groups of stem cells in contact that express pTMM:TMM-GFP . ( h ) Heat map images of pPIN3:PIN3-GFP and pDR5rev:3XVENUS-N7 in epidermis after dimethylsulphoxide (DMSO; mock) treatment. ( i ) NPA increases nuclear DR5 fluorescence in GMCs (arrows). ( j – o ) Time-lapse series showing NPA-induced excess unequal divisions in wild type. NPA significantly slows the decline of DR5 fluorescence in a new M (a white arrow); however, a M with high PIN3 levels progresses normally to stomatal differentiation (a green arrow). Scale bar, 10 μm. Full size image Pattern violations also appeared when auxin efflux was blocked chemically with 1-naphthylphthalamic acid (NPA) [27] . By contrast, patterning was unaffected by the application of native or synthetic auxin (IAA, NAA and 2,4-dichlorophenoxyacetic acid) or the auxin influx inhibitor (1-naphthoxyacetic acid) [28] , suggesting that intracellular auxin pools are tightly and locally regulated ( Fig. 2d,e ). TMM encodes a receptor-like protein that regulates stomatal production and patterning, and pTMM:TMM-GFP expression is specific to stomatal lineage cells [5] . NPA induced aggregations of small, TMM-GFP -positive stem cells in the epidermis, as well as mispatterned unequal divisions ( Fig. 2f,g ). NPA also prolonged the period of DR5 expression in GMCs ( Fig. 2h,i ) and extended the M to GMC auxin depletion phase (≥2.5 times, that is, 10.4±3.8–27.2±5.7 h; n =16–18, values are averages with s.d. ), but had little effect on DR5 expression in Ms with high PIN3 that divide unequally ( Fig. 2j–o , and Supplementary Fig. 7 and Supplementary Movie 4 ). Thus, high auxin efflux from Ms, for example, mediated by PIN3, is required for the M to GMC fate transition. Timely auxin depletion has also been shown to regulate seed dispersal [29] . Vesicular trafficking alters the stomatal division pattern Auxin function was also probed using the fungal toxin Brefeldin A (BFA) that disrupts PIN recycling, and thus auxin transport, by inhibiting ARF-GEF activity [30] , [31] . pGNOM:GNOM-GFP is widely expressed in the leaf epidermis. BFA (50 μM) induces subcellular aggregations of fluorescence from GNOM-GFP in cells in the stomatal lineage (as well as in other cell types). BFA treatment (60 min) induces PIN3-GFP internalization into the cell, an effect that was reduced after a 30-min water rinse ( Supplementary Fig. 8 ). BFA substantively increases stem cell proliferation in the stomatal pathway as well as misplaces unequal divisions that together lead to pattern violations ( Fig. 3a–j and Supplementary Figs 9 and 10 and Supplementary Movies 5 and 6 ). BFA also halves the number of precursor cells that exhibit differential PIN3 fluorescence ( Supplementary Table 1 ). Time-lapse microscopy after BFA treatment shows that DR5 levels drop in both sister cells and then lead to the abnormal formation of two stomata in contact ( Fig. 3k–o , and Supplementary Fig. 10 and Supplementary Movie 6 ). 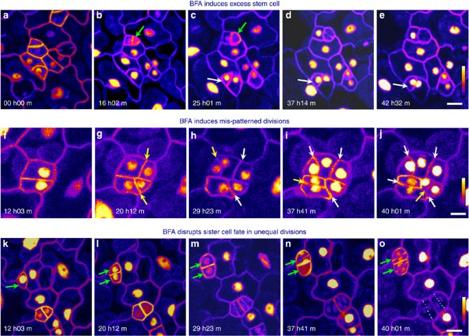Figure 3: Inhibition of vesicular trafficking alters the pattern of unequal and equal division. Heat map images ofpPIN3:PIN3-GFPandpDR5rev:3XVENUS-N7fluorescence in a BFA-treated epidermis viewed using time-lapse imaging. (a–e) BFA, like NPA, induces excessive unequal divisions and stem cells. DR5 fluorescence in a new M stays abnormally high (arrows). (f–j) BFA induces abnormal, excess and often adjacent unequal divisions of stomatal lineage stem cells. Each yellow arrow denotes a new unequal division; white arrows mark previous divisions. (k–o) BFA transforms divisions that are normally unequal in cell fate and size into equal ones. The M-like precursor cell (arrow ink) produces two daughter cells (paired arrows inl) with each forming a stoma. Scale bar, 10 μm. Figure 3: Inhibition of vesicular trafficking alters the pattern of unequal and equal division. Heat map images of pPIN3:PIN3-GFP and pDR5rev:3XVENUS-N7 fluorescence in a BFA-treated epidermis viewed using time-lapse imaging. ( a – e ) BFA, like NPA, induces excessive unequal divisions and stem cells. DR5 fluorescence in a new M stays abnormally high (arrows). ( f – j ) BFA induces abnormal, excess and often adjacent unequal divisions of stomatal lineage stem cells. Each yellow arrow denotes a new unequal division; white arrows mark previous divisions. ( k – o ) BFA transforms divisions that are normally unequal in cell fate and size into equal ones. The M-like precursor cell (arrow in k ) produces two daughter cells (paired arrows in l ) with each forming a stoma. Scale bar, 10 μm. Full size image Like pin mutants and NPA treatment, mutations in the BFA-sensitive ARF-GEF-encoding gene GNOM also disrupted stomatal patterning. The range of phenotypic severity of gnom alleles in stomatal formation was comparable to that previously shown in embryo and seedling development [32] , [33] . All gnom alleles (including gnom B/ E ) disrupted stomatal patterning, but the intermediate allele gnom R5 and the strong allele emb30-1 also induced swollen GCs ( Fig. 4a–c and Supplementary Fig. 11 ). Pattern defects were absent from plants treated with BFA but expressing an engineered BFA-resistant variant of GNOM ( Fig. 4d ), consistent with BFA inhibiting GNOM-mediated membrane trafficking including that of auxin transporters such as PIN3. Thus, GNOM-mediated trafficking controls stomatal morphogenesis as well as spacing. 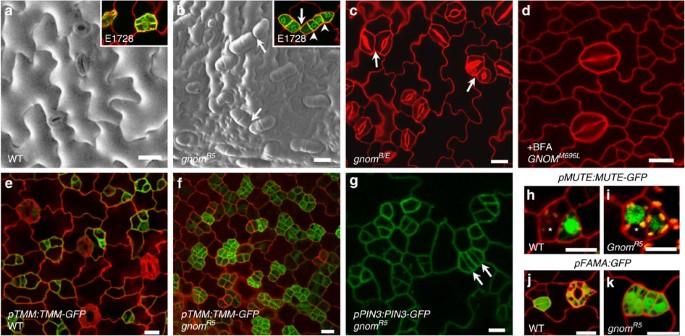Figure 4: GNOM is required for stomatal patterning and fate. (a) Cryo-scanning electron micrographs of wild-type epidermis. (b)gnommutant. Arrows, mispatterned and abnormally shaped GCs ingnomR5allele. Insets inaandbshow signal from the E1728, mature GC identity marker. (c)gnomB/E, a weaker allele, displays defects in patterning (arrows) but not morphogenesis. (d) BFA fails to disrupt patterning in BFA-resistant lineGNOMM696L. (e) Images of 2-day-old wild-type cotyledons. (f)gnomR5harbours abnormal groups ofTMM-expressing stem cells. (g) Excess small cells expressing bright PIN3 ingnomR5. Arrows, two developing stomata in contact. (h) Wild type showingpMUTE:MUTE-GFPexpression in the smaller cell (M) but not in its sister cell (asterisk). (i)gnomR5induces ectopicMUTEexpression in the larger daughter cell of unequal division (asterisk) next to its small sister cell. (j) Expression ofpFAMA:GFPis high in young wild-type GCs but is low in mature GCs. (k) Developing stomata in contact ingnomR5abnormally expresspFAMA:GFPin both sister cells. Scale bar, 10 μm. Figure 4: GNOM is required for stomatal patterning and fate. ( a ) Cryo-scanning electron micrographs of wild-type epidermis. ( b ) gnom mutant. Arrows, mispatterned and abnormally shaped GCs in gnom R5 allele. Insets in a and b show signal from the E1728, mature GC identity marker. ( c ) gnom B/E , a weaker allele, displays defects in patterning (arrows) but not morphogenesis. ( d ) BFA fails to disrupt patterning in BFA-resistant line GNOM M696L . ( e ) Images of 2-day-old wild-type cotyledons. ( f ) gnom R5 harbours abnormal groups of TMM- expressing stem cells. ( g ) Excess small cells expressing bright PIN3 in gnom R5 . Arrows, two developing stomata in contact. ( h ) Wild type showing pMUTE:MUTE-GFP expression in the smaller cell (M) but not in its sister cell (asterisk). ( i ) gnom R5 induces ectopic MUTE expression in the larger daughter cell of unequal division (asterisk) next to its small sister cell. ( j ) Expression of pFAMA:GFP is high in young wild-type GCs but is low in mature GCs. ( k ) Developing stomata in contact in gnom R5 abnormally express pFAMA:GFP in both sister cells. Scale bar, 10 μm. Full size image Pattern defects in gnom include groups of stomatal lineage-specific stem cells in contact as shown by pTMM:TMM-GFP fluorescence ( Fig. 4e,f ). A gnom tmm- double mutant showed a largely additive phenotype indicating that stomatal spacing arises via genetically distinct but functionally complementary pathways in which GNOM regulation of local auxin levels and TMM control of intercellular signalling orient adjacent unequal divisions ( Supplementary Fig. 12 ). BFA-induced pairs of stomata in contact were also found in gnom mutants ( Fig. 4g ). These pattern violations result from asymmetric divisions in which both sister cells express precursor cell genes ( MUTE and FAMA ) and then develop into stomata ( Fig. 4h–k ). Stomata form after at least one unequal division of a stem cell, and then by a single equal division of a GMC. Dynamic changes in auxin activity levels in stomatal development are represented by the auxin signalling input reporter 35 S:DII-VENUS-N7 , and by the output reporter pDR5rev:3XVENUS-N7 . High levels of fluorescence from the auxin efflux carrier PIN3 are present especially in the stomatal precursor cells, Ms and GMCs. Ms arise via an asymmetric division that is typically unequal in size as well as in cell fate. This division is usually preceded by nuclear migration towards the future division plane. Ms eventually acquire a GMC fate, a transition that requires MUTE. The larger sister cell produced by an unequal division can in turn function as an MMC by dividing asymmetrically thus producing a next-generation stoma. PIN3 levels increase slightly around the MMC before unequal division, and then decrease in the larger sister cell, but stay high throughout the lifespan of the M. PIN3 fluorescence levels peak in Ms and GMCs during the transition phase, whereas DR5 levels decrease during this developmental window. PIN3 levels also decrease during the symmetric division (of the GMC) as well as during stomatal morphogenesis ( Fig. 5 ). 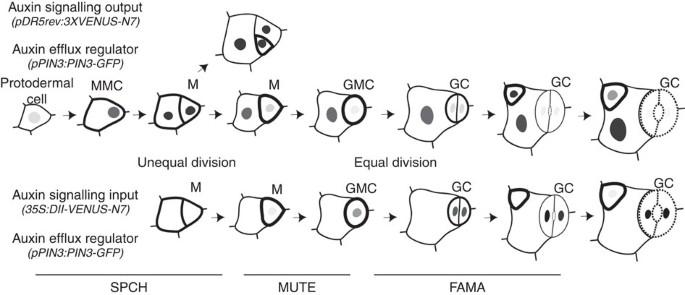Figure 5: Diagram of dynamics of auxin activity levels during stomatal development. Stomata develop after three fate transitions modulated by three sequentially acting bHLH transcription factors, SPEECHLESS (SPCH), MUTE and FAMA. Stomata form after at least one unequal division of a stem cell, and then by a single equal division of a GMC. Dynamic changes in auxin activity levels in stomatal development are represented by the auxin signalling input reporter35 S:DII-VENUS-N7(bottom row), and by the output reporterpDR5rev:3XVENUS-N7(top row). Relative fluorescence intensity levels are indicated in nuclei (circles or ovals) using a greyscale, with black maximal. Cell outlines indicate changes in the level of fluorescence from the PIN3 auxin efflux carrier with line thickness showing relative intensity levels. High levels are especially present in meristemoids (Ms) and guard mother cells (GMCs) that are stomatal precursors. Meristemoid mother cells (MMCs) arise from uncommitted protodermal cells via the action of SPCH. Ms originate in an asymmetric division that is usually unequal in size and fate. This division is usually preceded by nuclear migration towards the future division plane. Ms eventually acquire a GMC fate, a transition that requires MUTE. The larger sister cell produced by an unequal division can in turn function as an MMC by dividing asymmetrically thus producing a next-generation stoma. Larger sister cells of an asymmetric division that re-enter the stomatal cell lineage are termed stomatal lineage ground cells (SLGCs). PIN3 levels increase slightly around the MMC before unequal division, and then decrease in the larger sister cell, but stay high throughout the lifespan of the M. Peak levels of PIN3 fluorescence are present in Ms and GMCs, whereas DR5 levels decrease during the transition from M to GMC. PIN3 levels then decrease during the symmetric division (of the GMC) as well as during stomatal morphogenesis. Figure 5: Diagram of dynamics of auxin activity levels during stomatal development. Stomata develop after three fate transitions modulated by three sequentially acting bHLH transcription factors, SPEECHLESS (SPCH), MUTE and FAMA. Stomata form after at least one unequal division of a stem cell, and then by a single equal division of a GMC. Dynamic changes in auxin activity levels in stomatal development are represented by the auxin signalling input reporter 35 S:DII-VENUS-N7 (bottom row), and by the output reporter pDR5rev:3XVENUS-N7 (top row). Relative fluorescence intensity levels are indicated in nuclei (circles or ovals) using a greyscale, with black maximal. Cell outlines indicate changes in the level of fluorescence from the PIN3 auxin efflux carrier with line thickness showing relative intensity levels. High levels are especially present in meristemoids (Ms) and guard mother cells (GMCs) that are stomatal precursors. Meristemoid mother cells (MMCs) arise from uncommitted protodermal cells via the action of SPCH. Ms originate in an asymmetric division that is usually unequal in size and fate. This division is usually preceded by nuclear migration towards the future division plane. Ms eventually acquire a GMC fate, a transition that requires MUTE. The larger sister cell produced by an unequal division can in turn function as an MMC by dividing asymmetrically thus producing a next-generation stoma. Larger sister cells of an asymmetric division that re-enter the stomatal cell lineage are termed stomatal lineage ground cells (SLGCs). PIN3 levels increase slightly around the MMC before unequal division, and then decrease in the larger sister cell, but stay high throughout the lifespan of the M. Peak levels of PIN3 fluorescence are present in Ms and GMCs, whereas DR5 levels decrease during the transition from M to GMC. PIN3 levels then decrease during the symmetric division (of the GMC) as well as during stomatal morphogenesis. Full size image Collectively, our data show that PIN-mediated auxin depletion is required for a developmental switch in the cell lineage from unequal to equal division. The involvement of other auxin transport mechanisms such as ABCBs [16] and PIN-LIKES [34] in stomatal patterning cannot be excluded. Since BFA has also been shown to disrupt sterol trafficking [35] , it can not be ruled out that cell fate abnormalities are solely due to altered auxin transport, especially since the sterol pathway also regulates stomatal patterning [36] . In addition, auxin distribution and signalling restrict the size and promote the dispersion of the stomatal stem cell compartment. The respective functions and involvement of specific sets of PIN proteins, as well as of members of the TIR/AFB1 family, remained to be defined. Plant growth conditions and chemical treatment Seedlings were grown on half strength MS medium supplemented with 0.8% agar and 1% sucrose at 22–24 °C with an 8/16 h dark/light cycle. Chemical inhibitors were applied to seedlings grown for 2–3 days in multiple-well tissue culture plates. Microscopy Differential interference contrast images were obtained from living as well as cleared tissue. Propidium iodide (PI) staining of the epidermis was visualized using laser-scanning confocal microscopy. For time-lapse imaging, the adaxial cotyledon epidermis was then imaged every 6–9 h using a 40X water-dipping objective (Nikon CFI Fluor NA 0.8) and a Nikon C1 confocal microscope. Plant materials and phenotypic analysis The following Arabidopsis mutants and alleles were used in stomatal phenotype analysis. Single pin mutants/alleles were as follows: pin1-1 , pin2/ eir1-1 , pin3-5 , pin4-3 , pin5-5, pin6-2 , pin7-1 , pin8-1 . Double mutants were as follows: pin5-5 , 8-1 ; pin5-5 , 6-2 ; pin6-2, 8-1 ; pin3-5, 7EN ; pin3-5, 4-3 ; pin3-5, 1-1 ; pin4-3, 7-1 . Triple mutants were as follows: pin1-1, 4-3, 7-1 ; pin2-1, 3-5, 4-3 ; pin1-1, 2-1, 4-3 ; pin5-5, 6-2, 8-1 ; pin1-1, 3-5, 4-3 ; pin2-1, 3-5, 7-1 ; pin1-1, 3-5, 7-1 . Quadruple mutants were as follows: pin1-1, 3-5, 4-3, 7-1 ; pin2-1, 3-5, 4-3, 7-1 ; pin1-1, 2-1, 3-5, 7-1. Quadruple mutants related to auxin were as follows: tir1-1, afb1-1, 2-1, 3-1 (ref. 25 ) and tir1-1, afb1-3, 2-3, 3-4 (ref. 26 ). Since some mutant seedlings exhibit an array of different phenotypes, only seedlings lacking roots (class I) or with short roots (class II) [25] were used for stomatal phenotype assays. Similar stomatal patterning defects were found in pinoid-1 , which is a strong allele, but not in pinoid-2 or pinoid-3 (ref. 22 ). The detailed information of above mutants can be found in Supplementary Tables 2 and 3 . Expression patterns were analysed in young first leaves harbouring pPIN1:PIN1-GFP [37] , pPIN2:PIN2-GFP [37] , pPIN3:PIN3-GFP [17] , pPIN4:PIN4-GFP [24] , pPIN5:PIN5-GUS [38] , pPIN6:GUS [39] , pPIN7:PIN7-GFP [40] and pPIN8:PIN8-GFP [41] . The emb30-1 allele is a loss-of-function allele, whereas gnom R5 and gnom B/E are partial loss-of-function alleles [33] , [42] . The loss-of-function tmm-1 mutant, as well as the TMM translational GFP fusion ( pTMM:TMM-GFP ) were used [4] , [5] . E1728 is GAL4 GFP enhancer trap line used as a mature guard cell marker [43] . pMUTE:MUTE-GFP was used as a M/GMC marker [44] . Chemical treatment Seedlings were grown in multiple-well tissue culture plates for 2–3 days before covering with chemical solutions; all were obtained from Sigma–Aldrich. IAA, 1-naphthaleneacetic acid (NAA) and 2,4-dichlorophenoxyacetic acid were dissolved in ethanol and used at final concentrations of 50 and 20 μM, respectively. The auxin influx carrier inhibitor 1-naphthoxyacetic acid and the efflux carrier inhibitor NPA were dissolved in dimethylsulphoxide and used at a final concentration of 10 μM. Seedlings were immersed in chemical solutions for 1 day and then grown for 2–3 more days before stomatal phenotype analysis. GUS staining and imaging β-glucuronidase (GUS) assays and tissue clearing were performed as described [40] . Samples were mounted in 50% glycerol and imaged on an Olympus BX51 microscope. Cell outlines were visualized by staining with 0.5% PI for 1–2 min. Fluorescence from PI or fluorescent proteins was imaged using a Nikon C1 or an Olympus FV1000 confocal laser-scanning microscope. For cryo-scanning electron microscopy (SEM), cotyledons were dissected from soil-grown seedlings and mounted onto cryo-SEM stubs and plunged into liquid nitrogen. Frozen samples were transferred into an Emitech K1250 cryo-system and viewed with a Hitachi S4700 field emission SEM. Time-lapse imaging For time-lapse imaging, we used seedlings harbouring pPIN3:PIN3-GFP and either 35S:DII-VENU S-N7 (ref. 4 ) or pDR5rev:3XVENUS-N7 (ref. 5 ). Differentially high PIN3-GFP was separated from DR5 and background fluorescence signals by spectral linear unmixing. In addition, PIN3-GFP fluorescence can be distinguished from that of DR5 or DII by their cell membrane and nuclear localizations, respectively. Seedlings expressing PIN3-GFP and DR5/DII markers were grown on agar in small circular Petri dishes. Before imaging, dishes were attached to glass slides with Superglue (as well as stage clips) to hold them firmly on the microscope stage. Two to three-day-old cotyledons were placed on the surface of the agar, and the adaxial epidermis was imaged using a 40X water-dipping objective and a Nikon C1 confocal microscope. The x – y positions of the stage were recorded for each cotyledon, and then the entire Petri dish was returned to a growth chamber (22–24 °C and continuous light). Dishes were placed on the microscope stage every 6–9 h, and the same regions of the cotyledon were located by referring to x–y coordinates. For NPA or BFA treatment, drugs were applied directly to cotyledons. Fresh drug solutions were applied after each subsequent imaging. Image processing and analysis Spectral linear unmixing was accomplished using a Zeiss LSM 510 Meta Laser confocal scanning microscope. Seedlings harbouring either PIN3-GFP or DR5:VENUS , as well as wild-type controls with no marker genes, were used as individual controls. All microscope control settings, such as pinholes, gain, main beam splitter (HFT), detector range and microscope objectives, were identical for all the unmixing controls. The cell membranes of young seedlings harbouring pPIN3:PIN3-GFP were stained with 8 μM FM4-64 solution for 10 min before confocal imaging. The localization and intensity of FM-dyes and PIN3-GFP fluorescence were analysed with ImageJ (NIH, http://www.imagej.nih.gov/ij/ ) using Plot Profile. To test whether PIN3-GFP fluorescence was polarized in stomatal precursor cells, PIN3-GFP plot profiles along different transect lines in multiple directions were compared with those from FM-dyes fluorescence. Images of yz or xz sections of cells of interest were generated from confocal z-stacks using the orthogonal views function in ImageJ. To indicate fluorescence intensity using heat maps with a calibration bar, raw confocal images were converted into 8-bit grey value images before applying a Fire lookup table plugin installed in ImageJ software. To align time-lapse images, original confocal z-stacks were processed using the Maximum Intensity Projection function in ImageJ. The first time point was used as the target image, with subsequent images used as the source image in ImageJ with the TurboReg plugin ( http://www.bigwww.epfl.ch/thevenaz/turboreg ). The cursor was placed over the cell of interest, and then alignment direction was selected and subsequently applied to all other alignments. The new image generated from the previous source image was in turn used as the target image for aligning the image at the next time point. After aligning all images in the time window, the image from the first time point, as well as aligned images from subsequent times, were imported into ImageJ. The resulting image stacks were exported as AVI files with a playback rate of 1 frame per s. Quantification of changes in fluorescence levels Images from time-lapse series were scored using ImageJ software. DR5 activity was estimated by measuring the intensity of total nuclear fluorescence driven by the pDR5rev:3XVENUS-N7 construct. The sum of fluorescence intensity of DR5:VENUS was determined via optical sections (Z-projection function in ImageJ). Changes in the ratio of DR5:VENUS fluorescence during the M to GMC developmental transition that were greater than 1.5 were scored as a reduction in fluorescence. PIN3 expression levels were quantified by sampling average PIN3-GFP fluorescence intensity around the cell membrane. PIN3-GFP fluorescence ratios greater than 1.5 were scored as preferential expression in Ms and in GMCs as compared with their larger sister cell. Cells with a paradermal area similar to or lower than a normal GMC were classified as ‘small cells’ ( Supplementary Table 1 ). How to cite this article: Le, J. et al. Auxin transport and activity regulate stomatal patterning and development. Nat. Commun. 5:3090 doi: 10.1038/ncomms4090 (2014).